Dynamic analyses of alternative polyadenylation from RNA-seq reveal a 3′-UTR landscape across seven tumour types Alternative polyadenylation (APA) is a pervasive mechanism in the regulation of most human genes, and its implication in diseases including cancer is only beginning to be appreciated. Since conventional APA profiling has not been widely adopted, global cancer APA studies are very limited. Here we develop a novel bioinformatics algorithm (DaPars) for the de novo identification of dynamic APAs from standard RNA-seq. When applied to 358 TCGA Pan-Cancer tumour/normal pairs across seven tumour types, DaPars reveals 1,346 genes with recurrent and tumour-specific APAs. Most APA genes (91%) have shorter 3′-untranslated regions (3′ UTRs) in tumours that can avoid microRNA-mediated repression, including glutaminase ( GLS ), a key metabolic enzyme for tumour proliferation. Interestingly, selected APA events add strong prognostic power beyond common clinical and molecular variables, suggesting their potential as novel prognostic biomarkers. Finally, our results implicate CstF64 , an essential polyadenylation factor, as a master regulator of 3′-UTR shortening across multiple tumour types. The dynamic usage of messenger RNA (mRNA) 3′-untranslated region (3′ UTR), mediated through alternative polyadenylation (APA), plays an important role in post-transcriptional regulation under diverse physiological and pathological conditions [1] , [2] . Approximately 70% of human genes [3] are characterized by multiple polyA sites that produce distinct transcript isoforms with variable 3′-UTR length and content, thereby significantly contributing to transcriptome diversity [4] . The majority of APA examples utilize alternative polyA sites located within the terminal exon proximally downstream of the stop codon (tandem APA). As a result, while the protein-coding sequence is unaltered, the regulatory elements in the distal 3′ UTR that might reduce mRNA stability or impair translation efficiency can be removed, including AU-rich elements [5] and microRNA (miRNA)-binding sites [6] . A small percentage of APA sites can be located within internal introns/exons (splicing APA) and are coupled with alternative splicing to produce mRNA isoforms encoding distinct proteins. A well-documented example occurs during B-cell differentiation, where IgM switches from a membrane-bound form to a secreted form using a proximal polyA site instead of a distal one [7] . More recent studies [8] have shed light on the importance of APA in human diseases such as cancer, but its clinical significance to tumorigenesis is only beginning to be appreciated. Both proliferating cells [2] , [9] and transformed cells [10] have been shown to favour expression of shortened 3′ UTRs through APA, leading to activation of several proto-oncogenes, such as cyclin D1 (ref. 8 ). Collectively, these observations imply that truncation of the 3′ UTRs may serve as prognostic biomarkers [10] , [11] . While compelling, these studies were highly limited to either a limited number of genes or a small sample size. It remains to be determined to what extent APA occurs in cancer patients, what level of clinical utility APA may have and the molecular mechanisms and functional consequences of APA during tumorigenesis across multiple tumour types. RNA-seq has become a routine protocol for gene expression analysis; however, methods to quantify relative APA usage are still under development. Previous global APA studies use microarrays [2] , [12] , which are limited by the dependence on annotated polyA databases as well as inherent technical biases such as cross-hybridization. Recent APA protocols use polyA junction sites enrichment followed by high-throughput sequencing (PolyA-seq) [13] , [14] . These PolyA-seq protocols, although powerful in providing the precise locations of polyA sites, are hampered by technical issues, such as internal priming artefacts, and thus have not been widely adopted by the cancer community. In contrast, RNA-seq has been widely employed in almost every large-scale genomics project, including The Cancer Genome Atlas (TCGA). However, very few RNA-seq reads contain polyA tails, challenging our ability to identify APA events. For example, an ultra-deep sequencing study [15] only identified ~40 thousand putative polyA reads (~0.003%) from 1.2 billion total RNA-seq reads. Moreover, although the popular RNA-seq tool MISO [16] can detect annotated alternative tandem 3′ UTRs, it cannot identify any novel APA events beyond polyA databases. Finally, the short 3′ UTRs are often embedded within the long ones, and thus the isoforms with short 3′ UTRs are commonly overlooked by transcript assembly tools, such as Cufflinks [17] . Despite these inherent limitations, we hypothesize that any major changes in APA usage between different conditions will result in localized changes in RNA-seq density near the 3′-end of mRNA. And this localized RNA-density change can be readily detected through single-nucleotide resolution RNA-seq analysis. We therefore developed a novel bioinformatics algorithm, Dynamic analyses of Alternative PolyAdenylation from RNA-Seq (DaPars), to directly infer dynamic APA events through the comparison of standard RNA-seq data between different conditions. TCGA has characterized a comprehensive list of genomic, epigenomic and transcriptomic features in thousands of tumour samples; however, it lacks a PolyA-seq platform for APA analysis. To fill this knowledge gap, we used DaPars to retrospectively analyse the existing RNA-seq data of tumours and matched normal tissues derived from 358 patients across 7 tumour types. We discover 1,346 genes with highly recurrent tumour-specific dynamic APA events, demonstrate the additional prognostic power of APA beyond common clinical and molecular variables and expand our knowledge of the mechanisms and consequences of APA regulation during tumorigenesis. DaPars identifies dynamic APA events DaPars performs de novo identification and quantification of dynamic APA events between tumour and matched normal tissues, regardless of any prior APA annotation. For a given transcript, DaPars first identifies the de novo distal polyA site based on a continuous RNA-seq signal independent of the gene model ( Fig. 1a ; Supplementary Fig. 1a,b ). Assuming there is an alternative de novo proximal polyA site, DaPars models the normalized single-nucleotide resolution RNA-seq-read densities of both tumour and normal as a linear combination of both proximal and distal polyA sites. DaPars then uses a linear regression model to identify the location of the de novo proximal polyA site as an optimal fitting point (vertical arrow in Fig. 1a ) that can best explain the localized read-density change. Furthermore, this regression model is extended towards internal exons, so that splicing-coupled APA events can also be detected. Finally, the degree of difference in APA usage between tumour and normal can be quantified as a change in Percentage of Distal polyA site Usage Index (ΔPDUI), which is capable of identifying lengthening (positive index) or shortening (negative index) of 3′ UTRs. The dynamic APA events with statistically significant ΔPDUI between tumour and normal will be reported. The DaPars algorithm is described in further detail in the Methods. One example of an identified dynamic APA event is given for the TMEM237 gene ( Fig. 1b ), where the shorter 3′ UTR predominates in both breast (breast invasive carcinoma (BRCA)) and lung (lung squamous cell carcinoma (LUSC)) tumours compared with matched normal tissues. Another example is LRRFIP1 ( Fig. 1c ), where the distal 3′ UTR is nearly absent in both breast and lung tumours. 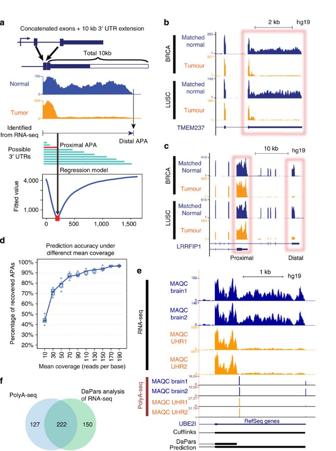Figure 1: Overview of the DaPars algorithm and its performance evaluation. (a) Diagram depicts the DaPars algorithm for the identification of dynamic APA between tumour and normal samples. The top panel shows RNA-seq coverage on exons with 10 kb extension without any prior knowledge of APA sites. The distal APA site is inferred directly from the combined RNA-seq data of tumour and normal tissues (middle panels). Theyaxis of the bottom panel is the fitted value of our regression model and the locus with the minimum fitted value (red point below vertical arrow) corresponds to the predicted proximal APA site (red horizontal bar). (b) An example of DaPars identified dynamic APA from the TCGA RNA-seq data. The shorter 3′ UTR ofTMEM237is preferred in BRCA and LUSC tumours. (c) Another example of dynamic APA, here the distal APA ofLRRFIP1is nearly absent in both BRCA and LUSC tumours while the proximal APA is unchanged. (d) A simulation study to demonstrate DaPars performance. The percentage of recovered APA events is plotted against different sequencing coverage. The quantile box shows the variation of DaPars prediction based on 1,000 simulated events. The black line in each box is the median recovery rate. (e) An example of dynamic APA between MAQC UHR and brain detected by both DaPars analysis of RNA-seq and PolyA-seq. The three bottom tracks are the RefSeq gene structure, Cufflinks prediction and DaPars prediction. (f) Venn diagram comparison between PolyA-seq and DaPars analysis of RNA-seq based on the same MAQC UHR and brain samples. Figure 1: Overview of the DaPars algorithm and its performance evaluation. ( a ) Diagram depicts the DaPars algorithm for the identification of dynamic APA between tumour and normal samples. The top panel shows RNA-seq coverage on exons with 10 kb extension without any prior knowledge of APA sites. The distal APA site is inferred directly from the combined RNA-seq data of tumour and normal tissues (middle panels). The y axis of the bottom panel is the fitted value of our regression model and the locus with the minimum fitted value (red point below vertical arrow) corresponds to the predicted proximal APA site (red horizontal bar). ( b ) An example of DaPars identified dynamic APA from the TCGA RNA-seq data. The shorter 3′ UTR of TMEM237 is preferred in BRCA and LUSC tumours. ( c ) Another example of dynamic APA, here the distal APA of LRRFIP1 is nearly absent in both BRCA and LUSC tumours while the proximal APA is unchanged. ( d ) A simulation study to demonstrate DaPars performance. The percentage of recovered APA events is plotted against different sequencing coverage. The quantile box shows the variation of DaPars prediction based on 1,000 simulated events. The black line in each box is the median recovery rate. ( e ) An example of dynamic APA between MAQC UHR and brain detected by both DaPars analysis of RNA-seq and PolyA-seq. The three bottom tracks are the RefSeq gene structure, Cufflinks prediction and DaPars prediction. ( f ) Venn diagram comparison between PolyA-seq and DaPars analysis of RNA-seq based on the same MAQC UHR and brain samples. Full size image DaPars evaluation using simulated and experimental APA data To assess the performance of DaPars, we conducted a series of proof-of-principle experiments. First, we used simulated RNA-seq data with predefined APA events to evaluate DaPars as a function of sequencing coverage. We simulated 1,000 genes in tumour and normal at different levels of sequencing coverage (reads per base gene model). For each gene, we simulated two isoforms with long and short 3′ UTRs (3,000 and 1,500 bp), respectively. The relative proportion of these two isoforms is randomly generated, so that the ΔPDUI between tumour and normal for each gene is a random number ranging from −1 to 1. According to these gene models and expression levels, we used Flux Simulator [18] to generate 50-bp paired-end RNA-seq reads with a 150-bp fragment length, taking into account typical technical biases observed in RNA-seq. The simulated RNA-seq reads were used as the input for DaPars analysis, while the short/long isoforms and the ΔPDUI values were hidden variables to be determined by DaPars. As a criterion for accuracy, the DaPars dynamic APA prediction is considered to be correct if the predicted de novo APA is within 50-bp distance of the bona fide polyA site, and the predicted ΔPDUI is within 0.05 from the pre-determined ΔPDUI. The final prediction accuracy (percentage of recovered APAs) is plotted as a function of the different coverage levels ( Fig. 1d ). Using genes with a single isoform as negative controls, we also reported receiver-operating characteristic curves at different coverage levels with areas under receiver-operating characteristic curves (AUCs) ranging from 0.762 to 0.985 ( Supplementary Fig. 2 ). Our results indicate that dynamic APA events can be readily identified across a very broad range of coverage levels. Importantly, we determined that a sequencing coverage of 30-fold can achieve >70% accuracy and close to 0.9 AUC in dynamic APA detection. Therefore, we filtered out genes with <30-fold coverage for all further analysis. As an additional proof-of-principle, we directly compared APA events detected by DaPars with that of PolyA-seq. To achieve this, we used the RNA-seq data [19] and PolyA-seq data [3] based on the same Human Brain Reference and the Universal Human Reference (UHR) MAQC samples [20] . For PolyA-seq, the differentially altered 3′-UTR usage was identified as described in Methods. From the comparison between brain and UHR, we found that ~60% ( P value<2.2e−16; Fisher’s exact test) of 372 DaPars predicted APA events could be strongly supported by PolyA-seq ( Fig. 1e,f ). Both PolyA-seq and DaPars reported longer 3′ UTRs in brain than in UHR in >94% dynamic APA events, which is consistent with recent reports that brain tissues normally have the longest 3′ UTRs [21] , [22] . Close inspection of the raw data indicates that the non-overlapping dynamic APA events can be partially explained by the individual assay limitations. For example, PolyA-seq is designed to amplify polyA tags; therefore, some dynamic APA events reported by PolyA-seq may have a small magnitude of changes that are not readily detectable by RNA-seq ( Supplementary Fig. 1c ). Meanwhile, probably due to additional steps such as fractionation, PolyA-seq may also fail to detect dynamic APAs that are clearly observed by RNA-seq ( Supplementary Fig. 1d ). Together, we conclude that DaPars can reliably detect dynamic APA events between different conditions using standard RNA-seq. Broad and recurrent shortening of 3′ UTRs across tumour types Since TCGA lacks a PolyA-seq platform for APA analysis, we sought to fill this knowledge gap through DaPars retrospective analysis of existing TCGA RNA-seq data, which were originally sequenced for gene expression. We focused our analysis on seven tumour types that have >10 tumour/normal pairs, including bladder urothelial carcinoma (BLCA), head and neck squamous cell carcinoma, LUSC, lung adenocarcinoma (LUAD), BRCA, kidney renal clear cell carcinoma (KIRC) and uterine corpus endometrioid carcinoma (UCEC) ( Supplementary Table 1 ). TCGA RNA-seq data are of high quality with a mean coverage of around 50-fold, which corresponds to 80% accuracy for DaPars APA analysis based on our simulation study ( Fig. 1d ). For each tumour type, we identified 224–744 genes with statistically significant and recurrent (occurrence rate >20%) dynamic APA events during tumorigenesis, leading to a total of 1,346 non-redundant events across 7 tumour types ( Fig. 2a ; Supplementary Fig. 3a ; Supplementary Data 1 ). As a negative control, we did not observe any recurrent APA events between different batches of normal tissues of the same tumour type, indicating that the 1,346 DaPars reported tumour-specific APA events are not likely due to technical artefacts, such as sequencing bias or batch effect. Overall, lung (LUSC and LUAD), uterine (UCEC), breast (BRCA) and bladder (BLCA) cancers possess the highest amount dynamic APA events than the other tumour types ( Fig. 2a ; Supplementary Fig. 3a,b ). Furthermore, 55% of the 1,346 dynamic APA events occur in at least 2 tumour types ( Supplementary Fig. 3c ), indicating potential concerted mechanisms in APA regulation across tumour types. Strikingly, the majority (61–98%) of APA events have shorter 3′ UTRs in tumours ( Fig. 2a ; Supplementary Fig. 3a ), which is consistent with previous reports that transformed cells preferentially express mRNAs with shortened 3′ UTRs [8] . 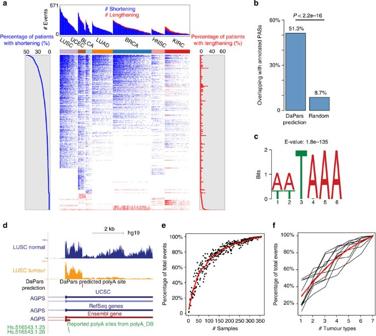Figure 2: Broad shortening of 3′ UTRs across seven TCGA tumour types. (a) The central heatmap shows genes (rows) undergoing 3′-UTR shortening (blue) or lengthening (red) in each of the 358 tumours (columns) compared with matched normal tissues across seven tumour types. The upper histogram shows the number of APA events per tumour. The side histograms show the percentage of tumours with 3′-UTR shortening (left) or lengthening (right) for each APA gene. (b) Bar plots show the percentages of DaPars-predicted APAs and randomly selected APAs from 3′-UTR regions overlapping with annotated APAs from four databases (Refseq, UCSC, ENSEMBL and PolyA_DB). ThePvalue was calculated byt-test using 50 × bootstrapping of data. (c) MEME identifies the canonical polyA motif AATAAA with a very significant E-value (1.8e−135) from the upstream (−50 bp) of the proximal polyA sites predicted by DaPars. (d) An example of DaPars-predicted novel polyA site (red bar) in a LUSC tumour that is far away from any annotated polyA sites. (e) Saturation analysis of APA events by adding more samples. Each point is a random subset of samples of various smaller sizes. All the points were fitted by a smoothed read line. (f) Saturation analysis by adding more tumour types. Each grey line represents a random ordering of seven tumour types and the red curve is the fitting line. The percentage of dynamic APA events increased with the number of tumour types. Figure 2: Broad shortening of 3′ UTRs across seven TCGA tumour types. ( a ) The central heatmap shows genes (rows) undergoing 3′-UTR shortening (blue) or lengthening (red) in each of the 358 tumours (columns) compared with matched normal tissues across seven tumour types. The upper histogram shows the number of APA events per tumour. The side histograms show the percentage of tumours with 3′-UTR shortening (left) or lengthening (right) for each APA gene. ( b ) Bar plots show the percentages of DaPars-predicted APAs and randomly selected APAs from 3′-UTR regions overlapping with annotated APAs from four databases (Refseq, UCSC, ENSEMBL and PolyA_DB). The P value was calculated by t -test using 50 × bootstrapping of data. ( c ) MEME identifies the canonical polyA motif AATAAA with a very significant E-value (1.8e−135) from the upstream (−50 bp) of the proximal polyA sites predicted by DaPars. ( d ) An example of DaPars-predicted novel polyA site (red bar) in a LUSC tumour that is far away from any annotated polyA sites. ( e ) Saturation analysis of APA events by adding more samples. Each point is a random subset of samples of various smaller sizes. All the points were fitted by a smoothed read line. ( f ) Saturation analysis by adding more tumour types. Each grey line represents a random ordering of seven tumour types and the red curve is the fitting line. The percentage of dynamic APA events increased with the number of tumour types. Full size image Multiple lines of evidence indicate that DaPars reported de novo APA events are indeed regulated through APA. First, 51% of DaPars predictions are within 50 bp of the annotated APAs compiled from Refseq, ENSEMBL, UCSC gene models and polyA database [23] . There is an approximately sixfold enrichment of annotated APAs in our DaPars predictions compared with random controls ( Fig. 2b ). Second, in the upstream (−50 nt) of our de nov APA sites, canonical polyA signal AATAAA can be successfully identified by MEME motif enrichment analysis [24] ( Fig. 2c ). In addition, AATAAA and ATTAAA are the most prevalent motifs among variants [25] of polyA signals ( Supplementary Fig. 4 ) [4] . By comparing ±50 bp flanking sequences of the distal and proximal polyA sites of the 3′-UTR shortening events, DREME [26] discriminative motif discovery algorithm reported that AATAAA motif is significantly stronger in distal polyA sites ( Supplementary Fig. 5 ), suggesting the molecular basis for differential polyA site selection [27] . Furthermore, the canonical polyA signal can also be identified ( Supplementary Figs 6 and 7 ) on those de novo APA sites that do not coincide with previous annotation. As expected, the de novo DaPars analysis enables us to detect novel APAs that are not annotated in any database. For example, we found a potential novel proximal APA site in AGPS that is significantly upregulated in LUSC tumour ( Fig. 2d ). Together, we conclude that DaPars reliably identified a comprehensive list of novel and existing APA target genes across seven TCGA tumour types, and the preferential shortening of 3′ UTR is a major layer of transcriptomic dynamics during tumorigenesis. APA events remain far from complete To explore to what extent the discovered 1,346 APA events have reached saturation, we performed ‘down-sampling’ saturation analysis. We repeated DaPars analysis (occurrence rate >20%) on random subsets of samples of various smaller sizes. Saturation is expected to occur when increasing sample size fails to discover additional APA events. The results indicate that the number of APA events increases steadily with increasing sample size in total ( Fig. 2e ), sample size per tumour type ( Supplementary Fig. 3d ) and the number of tumour types studied ( Fig. 2f ). This suggests that APA events derived from 358 samples across 7 tumour types remain far from complete. DaPars analysis on a larger sample size or more tumour types is likely to reveal many more novel APA events. This prediction is consistent with a recent report demonstrating that cancer genome sequencing normally requires thousands of samples per tumour type to approach saturation [28] . This observation also highlights the need for de novo discovery of APA, since any prior annotation-based detection methods are likely to miss a significant portion of novel APA events from tumour samples. Genes with shorter 3′ UTRs are prone to be upregulated The current model predicts that 3′-UTR shortening through APA during tumorigenesis may upregulate its parental gene by escaping miRNA repression. To test this hypothesis, we calculated the numbers of miRNA-binding sites lost due to 3′-UTR shortening in tumours ( Fig. 3a ). Using this approach, we determined that ~67% genes with shorter 3′ UTRs in tumours have lost at least 1 predicted miRNA-binding site ( Fig. 3a ). Furthermore, when compared with all the genes of sufficient sequencing coverage, those genes with shorter 3′ UTRs in tumours have overall greater miRNA-binding site density in their gene models ( P value=1.8e−11, t -test; Fig. 3b ). These data imply that APA regulation tends to maximize the miRNA-binding loss through preferentially shortening those 3′ UTRs already heavily regulated by miRNA. To examine the consequences of 3′ UTR and miRNA-binding loss, we compared the gene expression between tumours and matched normal tissues. As expected, those genes with shorter 3′ UTRs in tumours tend to be more upregulated in tumours ( Fig. 3c ). In conclusion, our data strongly support the hypothesis that many genes are upregulated during tumorigenesis by shortening their 3′ UTRs to escape post-transcriptional miRNA repression. 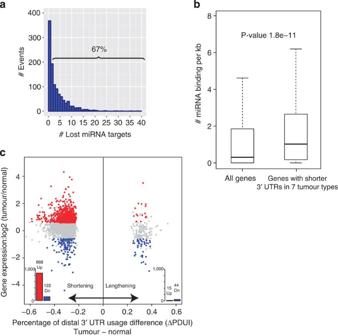Figure 3: Genes with shorter 3′ UTRs in tumours are prone to be upregulated. (a) Number of genes losing miRNA-binding sites due to the shortening of their 3′ UTRs. Here we selected miRNA-bindings sites predicted by both TargetScanHuman V6.2 (refs52,53) and miRanda54, as a more conservative list of miRNA targets. Number in the bracket represents the percentage of genes losing at least 1 miRNA-binding site. (b) Genes with shorter 3′ UTRs in tumours have greater miRNA-binding-site density in the 3′-UTR region than all RefSeq genes. We used RefSeq gene models for all the calculations regardless of the APA detection. Theyaxis is the number of miRNA-binding sites normalized by 3′-UTR length (per kb). ThePvalue was calculated by at-test. (c) For genes with shorter 3′ UTRs in tumours, their fold-change expression between tumours and normal tissues are plotted against their ΔPDUI values. All isoforms of the same gene were combined for the expression measurement. The genes significantly up- or downregulated in tumours are shown in red and blue, respectively, which were identified by pairedt-test with Benjamini–Hochberg (BH) false-discovery rate at 5%. Accordingly, the red and blue bar plots indicate the number of up- and downregulated genes, respectively. Figure 3: Genes with shorter 3′ UTRs in tumours are prone to be upregulated. ( a ) Number of genes losing miRNA-binding sites due to the shortening of their 3′ UTRs. Here we selected miRNA-bindings sites predicted by both TargetScanHuman V6.2 (refs 52 , 53 ) and miRanda [54] , as a more conservative list of miRNA targets. Number in the bracket represents the percentage of genes losing at least 1 miRNA-binding site. ( b ) Genes with shorter 3′ UTRs in tumours have greater miRNA-binding-site density in the 3′-UTR region than all RefSeq genes. We used RefSeq gene models for all the calculations regardless of the APA detection. The y axis is the number of miRNA-binding sites normalized by 3′-UTR length (per kb). The P value was calculated by a t -test. ( c ) For genes with shorter 3′ UTRs in tumours, their fold-change expression between tumours and normal tissues are plotted against their ΔPDUI values. All isoforms of the same gene were combined for the expression measurement. The genes significantly up- or downregulated in tumours are shown in red and blue, respectively, which were identified by paired t -test with Benjamini–Hochberg (BH) false-discovery rate at 5%. Accordingly, the red and blue bar plots indicate the number of up- and downregulated genes, respectively. Full size image APA events add prognostic power beyond common covariates Very little is known of the clinical implications of the dynamic 3′ UTRs in cancer patients. To address this issue, we used a standard Cox proportional hazards model [29] for the correlation between patient overall survival and multiple clinical and molecular covariates. Here we only used BRCA, LUSC and KIRC due to high mortality rate and large sample size. We first used common clinical covariates including only tumour stage, age, gender (excluding breast cancer) and smoking status (lung cancer only) to generate low- and high-risk groups, which are visualized by Kaplan–Meier plots and compared by the log-rank test ( Fig. 4a ). We next used the same Cox regression model integrated with LASSO to select the APA (ΔPDUI) events besides clinical covariates that can best separate risk groups. With clinical covariates always included, we used leave-one-out cross-validation (CV) to select the optimal 1–3 APA events ( Supplementary Table 2 ) to constitute new APA-clinical Cox regression models ( Fig. 4d ), which have much more significant P values in the risk group comparison. To quantify the added prognostic power of APA events, we used a likelihood-ratio test (LRT) to compare the new APA-clinical models with the clinical only models. The LRT results ( Fig. 4e ) clearly demonstrate a strong additional prognostic power of APA events beyond clinical covariates. Among these six APA covariates, significant worse survival is associated with 3′-UTR shortening of three genes ( SYNCRIP in BRCA; TMCO7 and PLXDC2 in KIRC) and 3′-UTR lengthening of two genes ( ATP5S in BRCA; RAB23 in LUSC) ( Supplementary Table 2 ). This result strongly suggests that, depending on the tumour types or genes studied, either lengthening or shortening of 3′ UTRs may be associated with poor clinical outcome. Since our CV procedure only selects the optimal APA events, it is highly likely that even more APA events can be associated with patient survival. Furthermore, we combined clinical covariates with tumour mRNA expression (mRNA-clinical) and tumour-vs-normal gene expression fold-change (mRNA-FC-clinical model) of the same APA genes ( Supplementary Table 2 ) as two additional Cox regression models and repeated the same analyses. Compared with the APA-clinical model, both mRNA-clinical and mRNA-FC-clinical models provide much less additional prognostic power ( Fig. 4e ), less-significant log-rank P values in risk group comparison ( Fig. 4b–d ). Finally, we show that the separated high- and low-risk groups by APA-clinical models have no correlation with the TCGA Pancan12 significantly mutated gene ( doi:10.7303/syn1750331 ) ( Fig. 4f ). Together, APA events provide additional power in survival prediction beyond clinical covariates, and independent of commonly used molecular data such as gene expression and somatic mutations. 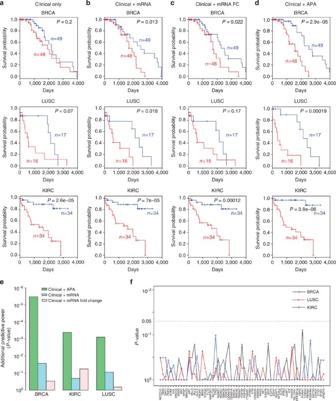Figure 4: Prognostic power of dynamic APA events. (a–d) Kaplan–Meier survival plots for high- (red line) and low (blue line)-risk groups separated by clinical only (a), clinical with mRNA expression (b), clinical with tumour-vs-normal mRNA expressions fold-change (c) and clinical with dynamic APAs (d).Pvalue was calculated using the log-rank test. (e) Additional prognostic power of APA, mRNA expression and mRNA tumour-vs-normal expression fold-change beyond clinical variables. ThePvalue is calculated by the likelihood-ratio test. (f) No correlation between risk groups separated by APA-clinical models and mutation profiles of significantly mutated genes (SMGs). The dotted vertical line represents thePvalue (Mann–Whitney test) cutoff of 0.05. All SMGPvalues are below this cutoff and thus are not significant. Figure 4: Prognostic power of dynamic APA events. ( a – d ) Kaplan–Meier survival plots for high- (red line) and low (blue line)-risk groups separated by clinical only ( a ), clinical with mRNA expression ( b ), clinical with tumour-vs-normal mRNA expressions fold-change ( c ) and clinical with dynamic APAs ( d ). P value was calculated using the log-rank test. ( e ) Additional prognostic power of APA, mRNA expression and mRNA tumour-vs-normal expression fold-change beyond clinical variables. The P value is calculated by the likelihood-ratio test. ( f ) No correlation between risk groups separated by APA-clinical models and mutation profiles of significantly mutated genes (SMGs). The dotted vertical line represents the P value (Mann–Whitney test) cutoff of 0.05. All SMG P values are below this cutoff and thus are not significant. Full size image Cancer metabolism gene GLS is regulated through APA Ingenuity IPA and literature searches were used to characterize the pathways enriched in 1,346 dynamic APA events ( Fig. 5a ; Supplementary Data 2 ). The vast majority of enriched pathways are cancer related, such as ERK/MAP signalling and glutamine metabolism. The metabolism gene glutaminase ( GLS ) is of particular interest. It is well known that tumours are considerably more dependent on the glycolytic pathway, regardless of oxygen availability, to supply a great deal of their energetic and biosynthetic demand for cell division. This phenomenon, termed the Warburg effect, is a hallmark of cancer [30] . GLS is a key enzyme in glutaminolysis and its high expression is essential to support the cancer metabolic phenotype [31] . There are two major GLS isoforms termed distal Kidney-type ( KGA ) and proximal Glutaminase C ( GAC ), which have distinct 3′ UTRs and slightly different C termini [32] , [33] , [34] ( Fig. 5b ). KGA has a number of miRNA-binding sites within its 3′ UTR, whereas GAC surprisingly is not predicted to have any ( Fig. 5b ). Furthermore, it has been shown that miR-23 represses KGA in most cells. However, in myc-transformed cells, MYC overexpression de-represses GLS through downregulation of miR-23 , resulting in glutamine-dependent growth characteristics [35] . Interestingly, we found a strong alternative-splicing-coupled 3′-UTR shift from KGA in normal to GAC in tumour, leading to a significantly increased percentage of GAC in LUAD, LUSC and KIRC ( Fig. 5b,c ). This is consistent with previous report that GAC is key to the mitochondrial glutaminase metabolism of cancer cells [31] . The implication of the 3′ UTR switch to GAC is that the expression of GLS is no longer regulated by miR-23 or MYC. Consistently, we did not observe any significant expression changes of miR-23 between tumours and normal tissues, although MYC is upregulated in LUSC and KIRC tumours ( Supplementary Fig. 8a ), suggesting that GLS potentially utilizes 3′-UTR switch, rather than MYC to escape miR-23 -mediated repression. 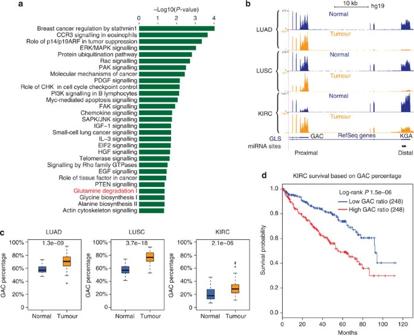Figure 5: Pathway analysis. (a) Significantly enriched (Pvalue<0.05; Fisher’s exact test) Ingenuity canonical pathways in the 1,346 dynamic APA events. (b)GLShas a significant 3′-UTR shift fromKGAlong isoform in normal toGACshort isoform in tumour. (c)GACpercentages are significantly higher in LUAD, LUSC and KIRC tumours. ThePvalue in each box was calculated using a pairedt-test. (d) Kaplan–Meier survival plot of two KIRC tumour groups stratified by the GAC ratios with equal patient number in each group.Pvalue was calculated using the log-rank test. Figure 5: Pathway analysis. ( a ) Significantly enriched ( P value<0.05; Fisher’s exact test) Ingenuity canonical pathways in the 1,346 dynamic APA events. ( b ) GLS has a significant 3′-UTR shift from KGA long isoform in normal to GAC short isoform in tumour. ( c ) GAC percentages are significantly higher in LUAD, LUSC and KIRC tumours. The P value in each box was calculated using a paired t -test. ( d ) Kaplan–Meier survival plot of two KIRC tumour groups stratified by the GAC ratios with equal patient number in each group. P value was calculated using the log-rank test. Full size image To investigate the potential clinical utility of the APA-mediated GLS isoform switch, we examined the correlation between GAC percentage and clinical survival information for KIRC tumours, using the Cox proportional hazards model with age and gender as covariates. We found that higher GAC percentage is highly correlated with worse survival ( P =3.2e−13, hazard ratio=50, 95% confidence interval: 17–141; Fig. 5d ), which is consistent with previous studies indicating that GAC is essential for cancer cell growth [36] . Overall, patients with high GAC ratios in KIRC have a median survival of ~55 months, compared with >92 months for those with low GAC ratios. We did not find a statistically significant correlation between GAC percentage and survival outcome in LUSC and LUAD possibly because the GAC percentages ((0.5, 0.97) and (0.59,0.98), respectively) ( Supplementary Fig. 8b ) have very limited dynamic range in these two tumour types, and thus may not have enough power to stratify patients. In contrast, GAC percentage ranges from 0.05 to 0.96 in KIRC ( Supplementary Fig. 8b ), allowing patient stratification based on a full range of GAC levels. Together, the GLS APA regulation suggests a novel and potentially MYC -independent and miRNA-independent mechanism of glutaminase regulation in tumours, and GLS APA can be used to predict patient survival in KIRC. Potential mechanisms for APA regulation during tumorigenesis We sought to investigate the potential mechanisms governing APA dynamics in tumorigenesis. Although many details remain poorly understood, APA is thought to be regulated in cis through genetic aberrations [37] , [38] of the underlying nascent mRNA (derived from DNA), and in trans by regulatory proteins in responding to dynamic environmental changes [39] . These cis -elements include canonical polyA signal AAUAAA and other auxiliary sequences such as U/GU-rich downstream elements [40] . The core polyadenylation trans -factors involve four multi-subunit protein complexes, CPSF (cleavage and polyadenylation specificity factor), CstF (cleavage stimulation factor), CFI and CFII (cleavage factors I and II). The chemical cleavage of pre-mRNA process mainly employs CPSF to recognize the canonical polyA signal upstream of the cleavage site, and utilizes CstF to bind downstream U/GU-rich elements [40] mainly through the CstF64 subunit [39] . To examine the role of genetic aberrations in the regulation of APA, we compared our 1,346 recurrent APA events with 64 Pancan12 Significantly Mutated Genes (doi:10.7303/syn1750331). Surprisingly, there are only five genes in common ( Fig. 6a ; P value 0.48 by Fisher’s exact test). This result indicates that most of the dynamic APA events are probably not due to aberrations of underlying cis -elements but may be the result of aberrant expression of polyA trans -factors. To address this possibility, we investigated the gene expression of 22 important polyA trans -factors [41] based on the TCGA RNA-seq data. The significantly up- and downregulated factors between tumours and matched normal tissues are indicated by yellow and blue, respectively ( Fig. 6b ). In general, we observed global upregulation of most polyA factors in five tumour types (LUSC, LUAD, UCEC, BLCA and BRCA), which also have more 3′-UTR-shortening events. Therefore, we conclude that most core polyadenylation factors are expressed at higher levels in tumour types where proximal APAs are favoured. Our results are consistent with previous studies showing that 3′-UTR shortening in proliferating cells is also accompanied by an increased expression of polyadenylation factors [9] , [12] , [27] . 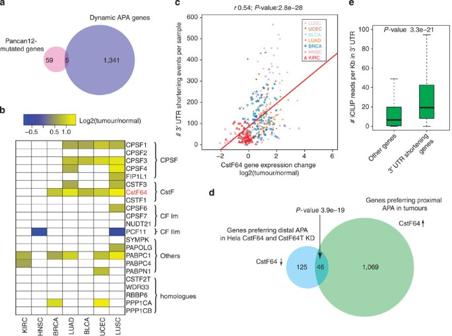Figure 6: Potential mechanisms for APA regulation during tumorigenesis. (a) Only five genes are in common between genes undergoing dynamic APA and genes significantly mutated in Pancan12 tumour types. (b) Heatmap of gene expression fold-change of known polyadenylation factors. Each rectangle represents the mean log2 fold-change between tumour and matched normal tissues of one factor in one tumour type. A factor is considered differentially expressed if the false-discovery rate from edgeR55is <0.05 and the mean absolute fold-change is >1.5. Yellow and blue boxes indicate the significantly upregulated and downregulated genes, respectively. White boxes are non-significant genes. (c) Correlation betweenCstF64expression fold-change and number of 3′-UTR-shortening events per sample. Each point represents a patient sample across seven tumour types. Thexaxis is theCstF64log2 fold-change between tumours and matched normal tissues. Theyaxis is the number of shortening events per sample. Spearman’s correlation coefficient (0.54) andPvalue (2.8e−28) are indicated on the top. (d) Venn diagram comparison between genes preferring proximal APAs in tumour with higher expression ofCstF64and genes preferring distal APA in Hela cells with knockdown ofCstF64andCstF64T. (e) Genes with 3′-UTR shortening in tumours have moreCstF64iCLIP data derived from HeLa cells than background (Pvalue 3.3e−21 byt-test). Figure 6: Potential mechanisms for APA regulation during tumorigenesis. ( a ) Only five genes are in common between genes undergoing dynamic APA and genes significantly mutated in Pancan12 tumour types. ( b ) Heatmap of gene expression fold-change of known polyadenylation factors. Each rectangle represents the mean log2 fold-change between tumour and matched normal tissues of one factor in one tumour type. A factor is considered differentially expressed if the false-discovery rate from edgeR [55] is <0.05 and the mean absolute fold-change is >1.5. Yellow and blue boxes indicate the significantly upregulated and downregulated genes, respectively. White boxes are non-significant genes. ( c ) Correlation between CstF64 expression fold-change and number of 3′-UTR-shortening events per sample. Each point represents a patient sample across seven tumour types. The x axis is the CstF64 log2 fold-change between tumours and matched normal tissues. The y axis is the number of shortening events per sample. Spearman’s correlation coefficient (0.54) and P value (2.8e−28) are indicated on the top. ( d ) Venn diagram comparison between genes preferring proximal APAs in tumour with higher expression of CstF64 and genes preferring distal APA in Hela cells with knockdown of CstF64 and CstF64T . ( e ) Genes with 3′-UTR shortening in tumours have more CstF64 iCLIP data derived from HeLa cells than background ( P value 3.3e−21 by t -test). Full size image We further investigated the correlation between gene expression and 3′-UTR shortening for four polyadenylation factors ( CPSF1 , CPSF3 , CstF64 and PABPC1 ), which are differentially expressed between tumour and normal in at least three cancer types ( Fig. 6b ). Among them, CstF64 has the greatest correlation between gene expression fold-change and the number of shortening events per patient in tumours (Spearman’s correlation 0.54 with P value 2.8e−28, Fig. 6c ), followed by CPSF3 . In contrast, CPSF1 and PABPC1 have weak correlations ( Supplementary Fig. 9 ). This result is consistent with a recent iClip-seq study, suggesting that CstF64 is one of the top three most important factors for polyA site selection [42] . Also, a recent study indicated that CPSF plays an important role in recruiting CstF64 to RNAs [43] . Furthermore, a recent global study in HeLa cells suggests that CstF64 induces the usage of proximal APAs [43] . They reported 171 genes with lengthening in 3′ UTRs upon knockdown of CstF64 , among which 46 genes from our analysis have shortened 3′ UTRs in tumours where CstF64 is upregulated ( Fig. 6d ; P value=3.9e−19 using Fisher’s exact test; Supplementary Fig. 10 ). This significant overlap indicates that a subset of 3′-UTR-shortening events we observed in tumours can indeed be explained by the expression level of CstF64 . Finally, using CstF64 iCLIP-seq in HeLa cells [43] , we showed that those 1,346 genes have more CstF64 bindings in their 3′ UTRs than other genes ( Fig. 6e ). Together, our study provides strong evidence that key polyA trans -factors, such as CstF64 , are upregulated in tumorigenesis, leading to preferential 3′-UTR shortening in tumours. We have developed a novel bioinformatics algorithm, termed DaPars, dedicated to the de novo identification and quantification of dynamic APA events using standard RNA-seq. The accuracy of DaPars is evidenced by the fact that our de novo predicted APAs are enriched for the canonical polyA signal AATAAA and have a high degree of overlap with annotated polyA sites ( Fig. 2b,c ). Our extensive DaPars analysis of TCGA data sets convincingly demonstrate that any investigator(s) conducting standard RNA-Seq is now capable of identifying the majority of functionally important APA events in most biological systems. DaPars is not just yet another APA assay; instead, its key methodology innovation is the inference of de novo APA events from existing RNA-seq data without relying on any additional wet-bench experiments. For example, our current APA analysis was based on RNA-seq of 358 tumour/normal pairs across 7 cancer types. An analysis of this scale would be prohibitively cumbersome using any previous method, such as microarrays, EST and PolyA-seq, but was made possible now with our DaPars method. While our paper was under review, Wang et al. [44] reported a change-point model to detect 3′-UTR switching using RNA-seq. The model by Wang et al. relies on the annotated distal polyA sites to infer the proximal ones, only supports genes with two polyA sites and only supports pair-wise comparison. In contrast, our DaPars method is fully de novo , can handle multiple (>2) polyA sites and multiple (>2) samples and thus is much more powerful and flexible than the model by Wang et al. . Most of our analyses based on hundreds of TCGA patient samples would not be possible using the model by Wang et al. It has been reported that shorter 3′ UTRs are preferentially used by several oncogenes in cancer cell lines [8] , but what was not clear from this work is how pervasive and recurrent APA is in clinical samples. Lin et al. [45] reported 126 3′-UTR-shortening genes in 5 tumour/normal pairs but unfortunately did not provide a supplementary table for those genes. To directly compare our results with Lin et al. [45] , we repeated the same analysis as described in their paper and detected a total of 120 genes with 3′-UTR shortening and upregulation of the short isoform. Among them, 53% were also found in our 1,201 shortening APA genes ( Supplementary Fig. 11 ; P value 2e−43 by Fisher’s exact test), including POLR2K , the main APA gene reported by Lin et al. Two examples of consistence and inconsistence between TCGA RNA-seq and PolyA-seq from Lin et al. [45] are shown in Supplementary Figs 12 and 13 , respectively. In this study, we have substantially increased the number of dynamic APA events based on 358 tumour/normal pairs. To our knowledge, this is the largest global APA analysis to date, leading to a 71-fold increase in sample size compared with Lin et al. [45] Several novel and significant biological and clinical insights are noticeable from our large-scale APA analysis. First, dynamic APA events are highly tumour type and patient specific. We observe that lung, uterus, breast and bladder cancers have significantly more APAs than head/neck and kidney cancers. Moreover, similar to other caner genomic data, there is considerable APA heterogeneity among patients within the same tumour type. Second, our saturation analysis indicates that APA events derived from 358 samples across 7 tumour types remain far from complete, highlighting the need for de novo discovery of APA, and the need for expanding DaPars analysis to more tumour types and samples when they become available. Third, selected APA events provide a surprisingly strong additional prognostic power beyond common clinical covariates and conventional molecular data, such as somatic mutation and gene expression. A recent study [46] also indicated that conventional molecular data had poor prognostic power beyond clinical data. Although the exact cause is unknown, we speculate that it may reflect a role for APA as a driver of tumour progression. Fourth, our study reveals a novel link between altered 3′-UTR usage and cancer metabolism. We observed that the GAC isoform of the glutaminase gene ( GLS ), which lacks any predicted miRNA binding, is predominantly expressed in LUSC, LUAD and KIRC tumours. Therefore, this APA event would abrogate the need to attenuate miR-23 expression through MYC upregulation and result in increased Glutaminase expression and altered glutamine metabolism. Fifth, our observation of correlating CstF64 levels with increased 3′-UTR shortening suggests that this factor is a potential master activator of proximal APA usage in tumorigenesis. This hypothesis predicts that tumour cells increase CstF64 levels to promote the 3′-end processing at the proximal and weaker polyA sites thereby preventing the usage of the distal polyA sites [39] , [43] . Finally, APA is likely to be regulated by many factors in a tissue-specific manner. For example, we recently reported CFIm25 (ref. 47 ) as a global repressor of proximal APA in brain tumour. CFIm25 has opposite function of CstF64, since its decreased expression correlates with increased 3′-UTR shortening. However, CFIm25 is not a master APA regulator in the cancer types we studied here, because it is not differentially expressed between tumour and normal ( NUDT21 in Fig. 6b ). Our DaPars analysis of RNA-seq reveals a comprehensive list of previously unobserved, highly recurrent and functionally important 3′-UTR somatic ‘RNA aberrations’. These RNA aberrations represent an illustrative case of genomic ‘dark matter’ beyond coding regions, and thus may also provide new directions for tumour gene discovery [48] . Although there is a lack in observed genetic aberrations within 3′ UTRs of most genes undergoing APA, caution should be taken as current TCGA mutation analyses utilize primarily exome sequencing, which excludes 3′ UTR. We will revisit this issue in the future when more whole-genome sequencing data are available. Finally, although focused on cancer genomics in this study, our novel DaPars framework will open the door for APA analysis in numerous biological and pathologic systems. It also underscores the power of innovative bioinformatics analyses that can derive novel biological insights from existing sequence data. Data sets All the RNA-seq BAM files were downloaded from the UCSC Cancer Genomics Hub (CGHub, https://cghub.ucsc.edu/ ). Here we only processed BRCA, BLCA, LUSC, LUAD, head and neck squamous cell carcinoma, UCEC and KIRC cancers that have >10 tumour–normal pairs ( Supplementary Table 1 ). Gene expression and miRNA expression were downloaded from The Cancer Genome Atlas data portal ( https://tcga-data.nci.nih.gov/tcga/dataAccessMatrix.htm ). MAQC brain and UHR RNA-seq reads were obtained from Sequence Read Archive with accessions ERP000016 and ERP000400, respectively. For MAQC PolyA-seq, the filtered polyA sites with normalized read counts were downloaded from the UCSC browser [3] . DaPars algorithm DaPars performs de novo identification and quantification of dynamic APA events between two conditions, regardless of any prior APA annotation. DaPars identifies a distal polyA site based on RNA-seq data, uses a regression model to infer the exact location of the proximal APA site after correcting the potential RNA-seq non-uniformity bias along gene body, detects statistically significant dynamic APAs and has the potential to detect >2 dynamic APA events. Distal polyA site identification from RNA-seq . Given two or more RNA-seq samples, distal polyA site refers to the end point of the longest 3′ UTR among all the samples, which will be used in the next step to identify the proximal polyA within this longest 3′-UTR region. To identify possible distal polyA site that may locate outside of gene annotation, we extend the annotated gene 3′ end by up to10 kb before reaching a neighbouring gene. RNA-seq data from all input samples will be merged to have a combined coverage along the extended gene model. To address possible uneven and discontinuous issues, we applied a 50-bp window to smooth this combined coverage. We then scan the extended 3′ UTR from 5′ to 3′ to find the distal polyA site whose coverage is significantly lower (that is,<predefined cutoff at 5%) than the coverage at the start of the preceding exon. A similar strategy has been successfully used to detect lengthening of 3′ UTRs in the mammalian brain [21] . The de novo distal APA estimated directly from RNA-seq, which may not be included in gene model, will benefit the downstream proximal APA identification ( Supplementary Fig. 1a ). Since most current RNA-seq data sets are not strand-specific, potential overlapping of 3′ UTRs from two neighbouring ‘tail-to-tail’ genes from different strands may give false-positive distal polyA. So after previous distal APA analysis, if 3′ UTRs of two neighbouring genes overlap, we will gradually increase the cutoffs until the two 3′ UTRs are separated. In this way, we can recover the proper distal polyA, which may be overlooked by other methods such as Cufflinks ( Supplementary Fig. 1b ). The distal polyA site identification method implemented in DaPars has very good performance. For all the predicted distal polyA sites from TCGA RNA-seq, on average 81% are within 50 bp of the annotated polyA sites. Regression model in DaPars . For each RefSeq transcript with a distal APA estimated from previous step, we use a regression model to infer the exact location of a de novo proximal polyA site at single-nucleotide resolution, by minimizing the deviation between the observed read density and the expected read density based on the two-polyA-site model, in both tumour and matched normal samples simultaneously. This regression model solves the following optimization problem: where and are the abundances of transcripts with distal and proximal polyA sites for sample i , respectively, C i =[ C i 1 ,···, C ij ,···, C iL ] T is the read coverage of sample i at single-nucleotide resolution normalized by total sequencing depth, L is the length of the longest 3′ UTR from previous step, P is the length of alternative proximal 3′ UTR to be estimated, I L and I P are indicator functions such that and . For each given 1< P < L , the expression levels of two transcripts with distal and proximal polyA sites in both tumour and normal tissues can be estimated by optimizing this linear regression model using quadratic programming [49] . The optimal de novo proximal polyA site P * is the one with the minimal objective function value, as demonstrated by the vertical arrow in Fig. 1a . To quantify the relative polyA site usage, we define the PDUI for sample i as the following: where and are the estimated expression levels of transcripts with distal and proximal polyA sites for sample i . The greater the PDUI is, the more distal polyA site of a transcript is used and vice versa. Finally, the regression model is extended towards the internal exons, so that splicing-coupled APA events can also be detected. Non-uniformity correction . It has been reported that RNA-seq reads are not uniformly distributed along the gene body. DaPars provides an option to address the issue of non-uniformity by statistical modelling [50] . Since it is technically difficult to distinguish non-uniform distribution from dynamic APA, we decide to train our statistical model based on a subset of genes with no APA change, that is, with only one 3′ UTR. We first run DaPars to select those genes with no APA change and divide their RNA-seq gene body coverage into 100 bins, yielding an observed gene body-sequencing profile ( Supplementary Fig. 1e ). In the conventional DaPars, the elements of I L and I P in equation (1) are unweighted and all 1s on 3′-UTR regions. We will infer the weighted I L and I P based on the observed gene body-sequencing profile, then re-run DaPars with the weighted I L and I P to correct the non-uniformity in RNA-seq ( Supplementary Fig. 1e ). Differential percentage of distal APA usage index . We used the following three criteria to detect the most significant APA events: first, given long 3′-UTR expression level and short 3′-UTR expression level estimated from (equation (1)), we used Fisher’s exact test to determine the P value of PDUI difference between tumour and matched normal tissue of the same patient, which is further adjusted by the Benjamini–Hochberg procedure to control the false-discovery rate (FDR) at 5%. Second, the absolute mean difference of PDUIs of all the patients in the same tumour type must be no less than 0.2. Third, the mean fold-change of PDUIs of all the patients in the same tumour type must be no less than 1.5. To avoid false-positive estimation on lowly expressed genes, we only included genes with >30-fold mean coverage (reads per base gene model). More than 2 dynamic APAs . Our DaPars framework can be easily extended to address >2 dynamic APAs. We formulated the multiple APA analysis in the following matrix format, where m is the length of the longest 3′ UTR of a transcript. w ij is the expression level of one possible 3′ UTR j on sample i . The number of non-zero w ij determines how many polyA sites will be derived from RNA-seq. In most cases, there are only a few w ij will be non-zero. So we can solve this equation using a positive Lasso optimization method as reformulated in the following form: where C , M and W are corresponding to the left, middle and right matrix in equation (4), respectively. In practice, we only consider no more than 4 APAs in a real data set to reduce the complexity of model selection and avoid over-fitting issues. In Supplementary Fig. 1f , we showed that our DaPars can also identify >2 APAs from RNA-seq and the predictions are highly consistent with the annotation. Although many genes have >2 annotated APAs, the majority of dynamic APAs only involve 2 polyA sites [1] . Therefore in the current large-scale TCGA RNA-seq analysis, we only focus on 2 APAs in the dynamic APA detection. PolyA-seq processing We downloaded the processed polyA sites with normalized read counts of MAQC brain and UHR PolyA-seq data sets (two replicates for each tissue) from the UCSC Genome Browser [3] . We calculated the signal intensity of a given polyA site based on all the same-strand PolyA-seq reads within 50 bases of the polyA site. We then used Fisher’s exact test to detect the statistically significant differential APAs between brain and UHR with a Benjamini–Hochberg-adjusted FDR cutoff of 0.1 and read count difference of >10%. For a fair comparison, we also used FDR of 0.1 and 10% ΔPDUI for DaPars analysis of MAQC RNA-seq data derived from the same brain and UHR samples. Survival analysis using Cox proportional hazards model A standard Cox proportional hazards model [29] implemented in the R package ‘survival’ was used for patient survival and Kaplan–Meier plotting. Hazard ratios exceeding 1 indicate poor prognosis for patients possessing shorter 3′ UTR, whereas those below 1 are associated with better outcome. The high-risk group and low-risk group were generated based on the prognostic index (PI). The PI is the linear component of the Cox model, where x i is the value of covariate i and its risk coefficient, β i was estimated from the Cox fitting. The high-risk and low-risk groups were generated for survival plot by splitting the ordered PI (higher values for higher risk) with equal number of samples in each group. Survival analysis using Cox model and LASSO feature selection We combined tumour-vs-normal shortening/lengthening events of APA genes (ΔPDUI values) with clinical covariates, such as age, gender, stage and smoking status (lung cancer), in survival analysis. We used a Cox regression model with LASSO feature selection to determine the contributions of APAs in survival prediction using the R package ‘glmnet’ [51] . We chose the optimal APA genes based on the leave-one-out CV. Here the clinical covariates are not penalized and always selected. Finally, we used a LRT to estimate the additional prediction power of the new APA-clinical models over the clinical-only models. Software availability The open source DaPars program is freely available at https://code.google.com/p/dapars/ . We will update this website periodically with new versions. How to cite this article: Xia, Z. et al. Dynamic analyses of alternative polyadenylation from RNA-seq reveal a 3′-UTR landscape across seven tumour types. Nat. Commun. 5:5274 doi: 10.1038/ncomms6274 (2014).